Notch2 activation ameliorates nephrosis Activation of Notch1 and Notch2 has been recently implicated in human glomerular diseases. Here we show that Notch2 prevents podocyte loss and nephrosis. Administration of a Notch2 agonistic monoclonal antibody ameliorates proteinuria and glomerulosclerosis in a mouse model of nephrosis and focal segmental glomerulosclerosis. In vitro , the specific knockdown of Notch2 increases apoptosis in damaged podocytes, while Notch2 agonistic antibodies enhance activation of Akt and protect damaged podocytes from apoptosis. Treatment with triciribine, an inhibitor of Akt pathway, abolishes the protective effect of the Notch2 agonistic antibody. We find a positive linear correlation between the number of podocytes expressing activated Notch2 and the number of residual podocytes in human nephrotic specimens. Hence, specific activation of Notch2 rescues damaged podocytes and activating Notch2 may represent a novel clinical strategy for the amelioration of nephrosis and glomerulosclerosis. Proteinuria and glomerulosclerosis are the major symptoms of glomerular diseases that have the risks to precede end-stage renal disease [1] , [2] . The number of the patients with end-stage renal disease is growing worldwide [3] , [4] , [5] , [6] . It is urgent to establish a new cure for glomerular diseases. Podocyte injury is a key factor of progression of glomerular damage detected in various glomerular diseases [7] . Continuous injury to podocytes induces podocyte loss, developing glomerulosclerosis. Therefore, inhibition of podocyte loss is of importance to prevent renal failure. Notch constitutes an evolutionarily conserved intercellular signalling pathway that determines cell fate in various organs [8] , [9] . This pathway is activated by interaction between Notch receptors and ligands between adjacent cells. On activation, Notch receptors are cleaved by γ-secretase and the intracellular domains translocate into the nucleus, where the transcription of target genes starts. There are four kinds of receptors (Notch1, Notch2, Notch3 and Notch4) and five ligands (Jagged1, Jagged2, DLL (Delta-like ligand)-1, DLL-3 and DLL-4) in mammalian organs. Notch pathways have pivotal roles in each stage during development [10] , [11] , [12] . In kidney, previous reports demonstrated that Notch1 and Notch2 were activated in mammalian nephrogenesis [10] , [11] . Afterward, Notch pathway becomes silent in matured glomeruli [12] , [13] . Niranjan et al . [14] recently reported that Notch1 was reactivated in kidney specimens of patients with diabetic nephropathy and with focal segmental glomerulosclerosis (FSGS) and that reactivation of Notch1 correlated with the development of proteinuria and glomerulosclerosis due to podocyte apoptosis in rodent models of glomerular disease. Since then, Notch pathway has attracted our attention as a target of new treatment. The existence of four Notch receptors suggests that each Notch receptor may have specific function. Notch1, but not Notch2, plays an essential role in T-cell development in the thymus [15] . In contrast, Notch2, but not Notch1, is essential for marginal zone B-cell development in the spleen [16] . Chen et al . [17] reported that only Notch2, but not Notch1, is required for the differentiation of proximal nephron structures. In mature kidney, Murea et al . [18] demonstrated that only reactivated Notch1 had a correlation with glomerulosclerosis in human glomerular diseases, while both Notch1 and Notch2 were reactivated. Thus, the function of reactivated Notch2 in glomerular diseases remains unclear. Here we demonstrate that activation of Notch2 with an agonistic monoclonal antibody (mAb) ameliorates proteinuria and glomerulosclerosis in mice with adriamycin (ADR)-induced nephropathy. In vitro , knockdown of Notch2 increases apoptosis in damaged podocytes and Notch2 agonistic mAb rescues podocytes from apoptosis through Akt pathway. Moreover, we find a positive linear correlation between activated Notch2 and podocyte preservation in human nephrotic specimens, suggesting the clinical utility of Notch2 agonists. Notch2 agonistic mAb ameliorates proteinuria in mice ADR nephropathy is a murine model of developing nephrosis and FSGS caused by podocyte injury [19] . We found that an injection of 10 mg kg −1 of ADR in mice induced significantly elevated proteinuria after 7 days, which peaked on day 14 ( Fig. 1a ). A previous report showed Notch activation in a diabetic mouse model and in puromycin aminonucleoside (PAN)-treated rats [14] . First, we examined the Notch activation in mice with ADR nephropathy. Immunofluorescent staining revealed increased expression of the active form of Notch1 (ICN1) and Notch2 (ICN2) in the nuclei of podocytes from 3 days after ADR injection ( Fig. 1b ). The strongest reactivation of Notch1 and Notch 2 occurred on day 7, the time point that coincides with the beginning of proteinuria ( Fig. 1b ). 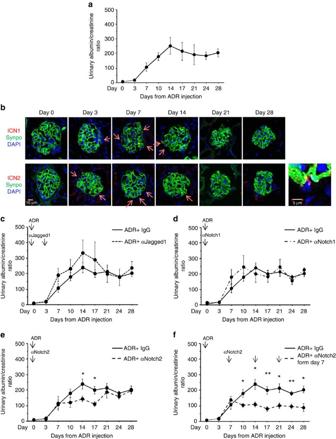Figure 1: Administration of Notch2 agonistic mAb ameliorates proteinuria in mice with ADR nephropathy. (a) Time course assessment of urinary albumin/creatinine ratio in mice with ADR nephropathy. A single dose (10 mg kg−1) of ADR was injected in mice via the tail vein on day 0. Urine samples were collected on the indicated days from at least five mice at each time point. (b) Cleaved Notch1 (ICN1; red in upper panels), cleaved Notch2 (ICN2; red in lower panels), synaptopodin (Synpo; green) and DAPI (blue) staining of kidney section of mice with ADR nephropathy at each time point. Red arrows indicate the expression of ICN1 and ICN2. Scale bar, 10 μm. Nuclear localization of ICN2 is represented at right. Scale bar, 5 μm. Jagged1 antagonistic mAb (αJagged1;c), Notch1 agonistic mAb (αNotch1;d) or Notch2 agonistic mAb (αNotch2;e) was intraperitoneally administered with the intravenous injection of ADR. (f) Notch2 agonistic mAb was intraperitoneally administered on 7, 14 and 21 days after the ADR injection. All the urine samples were collected on the indicated days and urinary albumin/creatinine ratios were measured. Data are indicated as the mean±s.e.m. of at least five mice in each group. *P<0.05, **P<0.01, Student’st-test. Figure 1: Administration of Notch2 agonistic mAb ameliorates proteinuria in mice with ADR nephropathy. ( a ) Time course assessment of urinary albumin/creatinine ratio in mice with ADR nephropathy. A single dose (10 mg kg −1 ) of ADR was injected in mice via the tail vein on day 0. Urine samples were collected on the indicated days from at least five mice at each time point. ( b ) Cleaved Notch1 (ICN1; red in upper panels), cleaved Notch2 (ICN2; red in lower panels), synaptopodin (Synpo; green) and DAPI (blue) staining of kidney section of mice with ADR nephropathy at each time point. Red arrows indicate the expression of ICN1 and ICN2. Scale bar, 10 μm. Nuclear localization of ICN2 is represented at right. Scale bar, 5 μm. Jagged1 antagonistic mAb (αJagged1; c ), Notch1 agonistic mAb (αNotch1; d ) or Notch2 agonistic mAb (αNotch2; e ) was intraperitoneally administered with the intravenous injection of ADR. ( f ) Notch2 agonistic mAb was intraperitoneally administered on 7, 14 and 21 days after the ADR injection. All the urine samples were collected on the indicated days and urinary albumin/creatinine ratios were measured. Data are indicated as the mean±s.e.m. of at least five mice in each group. * P <0.05, ** P <0.01, Student’s t -test. Full size image Jagged1 is a ligand of Notch pathway and has been reported to interact with both Notch1 and Notch2 (Oda et al . [20] and Shimizu et al . [21] ). To examine whether a blockade of Notch pathway has a protective effect on proteinuria in mice with ADR nephropathy, we administered an antagonistic mAb against Jagged1 intraperitoneally on days 0 and 3 after ADR injection. We found that anti-Jagged1 mAb tended to rather exacerbate proteinuria in mice with ADR nephropathy, although statistically insignificant ( Fig. 1c ), suggesting a protective role of Notch pathway. We then examined whether the acceleration of Notch pathway by agonistic mAb against Notch1 or Notch2 could improve the proteinuria in mice with ADR nephropathy. Administration of Notch1 agonistic mAb did not improve the proteinuria consistently ( Fig. 1d ). On the other hand, Notch2 agonistic mAb significantly decreased the levels of proteinuria from 14 days after ADR injection ( Fig. 1e ; P =0.039 at day 14 and P =0.0110 at day 17, Student’s t -test). Moreover, the ADR-induced proteinuria was markedly ameliorated when Notch2 agonistic mAb was therapeutically administered once a week from day 7 after ADR injection ( Fig. 1f ; P =0.0325, 0.0125, 0.0044, 0.0172, 0.0051 and 0.0271 at days 7, 10, 14, 17, 21 and 28, respectively, Student’s t -test). These results indicate that Notch2 agonistic mAb has a protective effect against proteinuria in mice with ADR nephropathy, even after the mice developed proteinuria. Notch2 pathway acceleration reduces glomerulosclerosis As we previously reported, ADR injection induces podocyte apoptosis in mice, resulting in podocyte loss and glomerulosclerosis [22] . We then assessed the effect of Jagged1 antagonistic mAb, Notch1 agonistic mAb and Notch2 agonistic mAb on glomerulosclerosis. Renal histology revealed glomerulosclerosis in the ADR-injected mice. In contrast, the mice injected with both ADR and Notch2 mAb showed less glomerular changes ( Fig. 2a ). The ratio of sclerotic glomeruli on day 28 was significantly decreased when Notch2 agonistic mAb was injected once on day 0 or three times on day 7, 14 and 21 compared with those when control IgG was injected once on day 0 ( P =0.0020 and P =0.0002, respectively, Student’s t -test), whereas it was increased when Jagged1 antagonistic mAb was injected ( P =0.0007, Student’s t -test; Fig. 2b ). Immunofluorescence study demonstrated the decreased number of WT1-positive cells on day 28 in mice with ADR nephropathy. In contrast, WT1-positive cells were mostly preserved when Notch2 agonistic mAb was administered in mice with ADR nephropathy ( P =0.0118 and P =0.0226, respectively, Student’s t -test; Fig. 2c ). These results indicate that Notch2 agonistic mAb prevented the podocyte loss and glomerulosclerosis as well as the proteinuria. Notably, these effects were observed not only when Notch2 agonistic mAb was administered simultaneously with ADR but also when the mAb was used therapeutically from day 7. 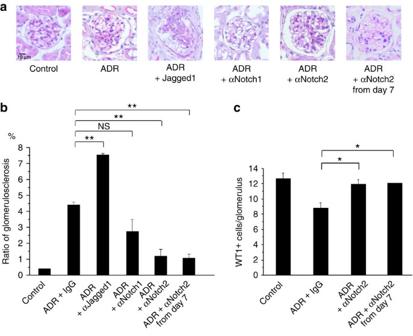Figure 2: Notch2 agonistic mAb preserves podocytes and suppresses the progression of glomerulosclerosis. Each group of mice was assessed: naive (control), ADR-injected, ADR and Jagged1 antagonistic mAb-injected (ADR+αJagged1), ADR and Notch1 agonistic mAb-injected (ADR+αNotch1), ADR and Notch2 agonistic mAb-injected (ADR+αNotch2) and Notch2 agonistic mAb-injected from 7 days after ADR injection (ADR+αNotch2 from day 7) as inFig. 1c–f. (a) Periodic acid–Schiff staining of representative kidney sections from each group. Scale bar, 10 μm. (b) The ratio of glomerulosclerosis was calculated by the proportion of the number of glomeruli with sclerosis to the number of total glomeruli. Data are presented as the means±s.e.m. of four to five mice in each group. **P<0.01. Student’st-test. The ratio of glomerulosclerosis in ADR+αJagged1 is significantly high, and the ratios of glomerulosclerosis in ADR+αNotch2 and in ADR+αNotch2 from day 7 are significantly low. (c) The number of podocytes in glomeruli of ADR+αNotch2 on day 28 was counted as WT1-positive cells, after triple staining of WT1, Synpo and DAPI. Data are presented as the means±s.e.m. of four to five mice in each group. Podocytes in ADR+αNotch2 and in ADR+αNotch2 from day 7 are significantly preserved. *P<0.05. Student’st-test. NS, not significant. Figure 2: Notch2 agonistic mAb preserves podocytes and suppresses the progression of glomerulosclerosis. Each group of mice was assessed: naive (control), ADR-injected, ADR and Jagged1 antagonistic mAb-injected (ADR+αJagged1), ADR and Notch1 agonistic mAb-injected (ADR+αNotch1), ADR and Notch2 agonistic mAb-injected (ADR+αNotch2) and Notch2 agonistic mAb-injected from 7 days after ADR injection (ADR+αNotch2 from day 7) as in Fig. 1c–f . ( a ) Periodic acid–Schiff staining of representative kidney sections from each group. Scale bar, 10 μm. ( b ) The ratio of glomerulosclerosis was calculated by the proportion of the number of glomeruli with sclerosis to the number of total glomeruli. Data are presented as the means±s.e.m. of four to five mice in each group. ** P <0.01. Student’s t -test. The ratio of glomerulosclerosis in ADR+αJagged1 is significantly high, and the ratios of glomerulosclerosis in ADR+αNotch2 and in ADR+αNotch2 from day 7 are significantly low. ( c ) The number of podocytes in glomeruli of ADR+αNotch2 on day 28 was counted as WT1-positive cells, after triple staining of WT1, Synpo and DAPI. Data are presented as the means±s.e.m. of four to five mice in each group. Podocytes in ADR+αNotch2 and in ADR+αNotch2 from day 7 are significantly preserved. * P <0.05. Student’s t -test. NS, not significant. Full size image Notch2 agonistic mAb protects podocytes from apoptosis To use cultured podocytes to assess the functions of Notch pathway, we examined the expression of Notch receptors (Notch1, Notch2, Notch3 and Notch4) and ligands (Jagged1, Jagged2, DLL-1 and DLL-4) on the surface of cultured podocytes by flow cytometry. We detected Notch2 receptor and Jagged1 ligand on the surface of cultured podocytes ( Supplementary Fig. 1a ). Next, we examined the induction of Notch ligands, which possibly interact with Notch2, on the surface of podocytes at 90 min after treatment with ADR. We detected only increased expression of Jagged1 ligand ( Supplementary Fig. 1b ), indicating that ADR could trigger Jagged1–Notch2 pathway. To explore the specific function of Jagged1–Notch2 pathway in podocytes, we treated cultured podocytes with ADR in the presence or absence of Notch2 agonistic mAb. We added 0.25 μg ml −1 of ADR to cultured podocytes to induce cell damage and examined the activation of Notch2 pathway. In western blotting, expression of both Notch2 and Jagged1 increased at 30–120 min after ADR treatment. Expression of cleaved Notch2, representing Notch2 activation, gradually increased from 30 min, which paralleled with the appearance of Jagged1. It peaked at 90 min, and disappeared at 150 min, which paralleled with the disappearance of Jagged1 ( Fig. 3a ). This suggests that ADR triggers Notch2 pathway activation in podocytes by induction of both Notch2 and Jagged1. Next, we examined the effect of Notch2 agonistic mAb on the ADR-induced Notch2 activation. The increase of cleaved Notch2 in ADR-treated podocytes was significant as compared with untreated control podocytes ( P =0.0009, Student’s t -test; Fig. 3b ). The expression of cleaved Notch2 markedly increased when Notch2 agonistic mAb was added ( Fig. 3b ; P <0.0001 as compared with ADR+IgG, Student’s t -test). Total Notch2, sum of cleaved Notch2 and full-length Notch2, was increased as well when podocytes were treated with ADR and control IgG (ADR+IgG), or ADR and Notch2 agonistic mAb (ADR+αNotch2; Supplementary Fig. 2 ; P =0.0407, Student’s t -test). This suggests that acceleration of Notch2 activation induces Notch2 expression. γ-secretase inhibitor (GSI) blocks the activation of canonical Notch pathway by preventing the cleavage of Notch receptor. Adding GSI to ADR-treated podocytes in the presence of Notch2 agonistic mAb abolished the increase of cleaved Notch2 ( Fig. 3b ), indicating that Notch2 agonistic mAb activates Notch2 by directly inducing cleavage of Notch2. We also assessed the messenger RNA expression in ADR-treated podocytes when control IgG or Notch2 agonistic mAb was added. As shown in Fig. 3c , mRNA expression of neither Jagged1 nor Notch2 was increased at 30 min after treatment when both Jagged1 and Notch2 proteins were increased ( Fig. 3a ). These results indicate that the expression of Jagged1 and Notch2 was upregulated at a post-transcriptional level. We also examined mRNA expression of Notch target genes ( Hes1 , Hes5 , Hey1 and HeyL ) at 6 h after treatment with ADR, ADR and Jagged1 antagonistic mAb, or ADR and Notch2 agonistic mAb. Compared with untreated control podocytes, Hes5 and Hey1 were increased but Hes1 and HeyL were decreased in ADR-treated podocytes ( Supplementary Fig. 3 ). Treatment of ADR-treated podocytes with Jagged1 antagonistic mAb abrogated the increase of Hes5 and Hey1, indicating the critical contribution of Jagged1. Interestingly, when Notch2 agonistic mAb was added simultaneously with ADR, Hes5 and Hey1 were suppressed and HeyL was recovered. 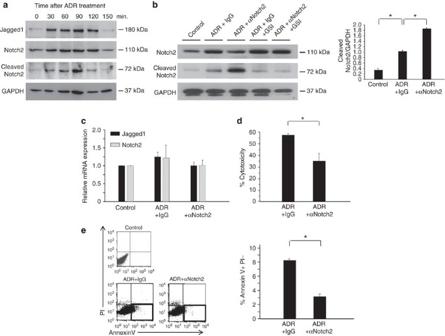Figure 3: Notch2 is activated in ADR-treated cultured podocytes and Notch2 agonistic mAb rescues damaged podocytes from apoptosis. Cultured podocytes were treated with 0.25 μg ml−1of ADR to induce cell damage. (a) Time course of the expression of Jagged1, Notch2 and cleaved Notch2 in ADR-treated podocytes were assessed by western blotting. (b) Western blotting analysis of the effects of Notch2 agonistic mAb (αNotch2) or control hamster IgG (IgG) on the expression of Notch2 and cleaved Notch2 in ADR-treated podocytes (left) with/without 10 μM γ-secretase inhibitor (GSI; left). Quantitative data of cleaved Notch2/GAPDH are shown (right). Data are represented as the means±s.e.m. (n=3). **P<0.001. Student’st-test. (c) Relative mRNA expression of Jagged1 and Notch2 at 30 min after treatment with Notch2 agonistic mAb (αNotch2) or control hamster IgG (IgG). Data are represented as the means±s.e.m. (n=3). (d) The percentages of cytotoxicity at 48 h after the ADR treatment were assessed by the LDH release assay. Data are represented as the means±s.e.m. of triplicated cultures. *P<0.05, Student’st-test. (e) Podocytes at 8 h after the ADR treatment were stained with APC-Annexin V/PI and analysed by flow cytometry (left). Percentages of Annexin V+ PI− apoptotic cells are indicated as the means±s.e.m. of triplicated cultures (right). *P<0.0001, Student’st-test. Figure 3: Notch2 is activated in ADR-treated cultured podocytes and Notch2 agonistic mAb rescues damaged podocytes from apoptosis. Cultured podocytes were treated with 0.25 μg ml −1 of ADR to induce cell damage. ( a ) Time course of the expression of Jagged1, Notch2 and cleaved Notch2 in ADR-treated podocytes were assessed by western blotting. ( b ) Western blotting analysis of the effects of Notch2 agonistic mAb (αNotch2) or control hamster IgG (IgG) on the expression of Notch2 and cleaved Notch2 in ADR-treated podocytes (left) with/without 10 μM γ-secretase inhibitor (GSI; left). Quantitative data of cleaved Notch2/GAPDH are shown (right). Data are represented as the means±s.e.m. ( n =3). ** P <0.001. Student’s t -test. ( c ) Relative mRNA expression of Jagged1 and Notch2 at 30 min after treatment with Notch2 agonistic mAb (αNotch2) or control hamster IgG (IgG). Data are represented as the means±s.e.m. ( n =3). ( d ) The percentages of cytotoxicity at 48 h after the ADR treatment were assessed by the LDH release assay. Data are represented as the means±s.e.m. of triplicated cultures. * P <0.05, Student’s t -test. ( e ) Podocytes at 8 h after the ADR treatment were stained with APC-Annexin V/PI and analysed by flow cytometry (left). Percentages of Annexin V+ PI− apoptotic cells are indicated as the means±s.e.m. of triplicated cultures (right). * P <0.0001, Student’s t -test. Full size image To determine whether Notch2 agonistic mAb has a protective effect against ADR-induced podocyte injury, we examined cytotoxicity by lactate dehydrogenase (LDH) release assay at 48 h after ADR treatment with or without Notch2 agonistic mAb. Cultured podocytes treated with ADR showed more than 50% of cytotoxicity at 48 h, which was significantly reduced by the addition of Notch2 agonistic mAb ( Fig. 3d ). We also examined apoptosis of ADR-treated podocytes by the annexin V/propidium iodide (PI) staining method. As shown in Fig. 3e , ADR-treated podocytes contained substantial percentages of apoptotic cells (6.65±1.62%, the mean±s.e.m. ), which was significantly reduced by Notch2 agonistic mAb (3.15±0.34%, the mean±s.e.m.). These results indicate that Notch2 agonistic mAb protects ADR-damaged podocytes from apoptotic cell death. Notch2 plays a critical role in podocyte survival While Notch2 agonistic mAb reduced apoptosis of ADR-treated podocytes as shown in Fig. 3e , GSI abolished the protective effect of Notch2 agonistic mAb ( P =0.0003, Student’s t -test; Fig. 4a ). This indicates that the canonical Notch2 signalling is responsible for the protection. To confirm the anti-apoptotic function of Notch2, we generated Notch2-knockdown (N2KD) podocytes by transduction of three different lentiviral vectors expressing Notch2 short hairpin RNA (shRNA) and GFP (N2KD-1, N2KD-2 and N2KD-3). Every N2KD podocytes showed significantly reduced Notch2 expression as compared with the non-silencing shRNA-transduced podocytes (control; Fig. 4b ). Next, we examined apoptosis of N2KD podocytes injured by ADR. As shown in Fig. 4c , the ratio of apoptotic cells in each N2KD podocytes was significantly elevated in the N2KD podocytes as compared with the control ( P =0.0064, P =0.0105 and P =0.0038 in N2KD-1, N2KD-2 and N2KD-3, respectively, Student’s t -test). These results indicate that Notch2 plays a critical role in protecting injured podocytes from apoptosis. 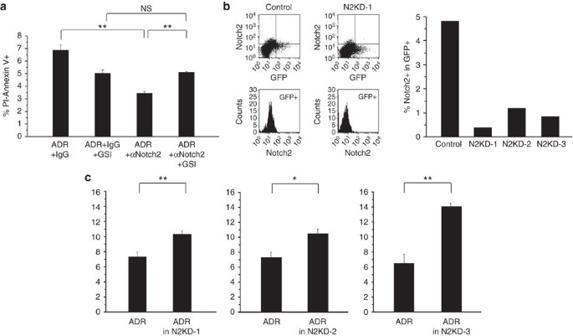Figure 4: Notch2 inhibition or knockdown increases ADR-induced podocyte apoptosis. (a) Percentages of apoptotic podocytes treated with ADR and control hamster IgG (IgG) or Notch2 agonistic mAb (αNotch2) in the absence or presence of γ-secretase inhibitor (GSI). Data are represented as the means±s.e.m. (n=4 or 5). *P<0.05, **P<0.01, Student’st-test. (b) Flow cytometry in the left panels shows expression of green fluorescent protein (GFP) and Notch2 in cultured podocytes transduced with non-silencing shRNA (control) or three Notch2 shRNAs (N2KD-1, 2, 3). Notch2 expression on the GFP+-transduced cells are indicated as histograms in the lower panels. Percentages of Notch2+ cells in GFP+ cells are also shown (right). (c) The podocytes transduced with control shRNA or Notch2 shRNAs were treated with 0.25 μg ml−1of ADR for 8 h. Percentages of Annexin V+ apoptotic cells in GFP+-transduced cells are indicated as the means±s.e.m. of triplicated cultures. **P<0.01, Student’st-test. Figure 4: Notch2 inhibition or knockdown increases ADR-induced podocyte apoptosis. ( a ) Percentages of apoptotic podocytes treated with ADR and control hamster IgG (IgG) or Notch2 agonistic mAb (αNotch2) in the absence or presence of γ-secretase inhibitor (GSI). Data are represented as the means±s.e.m. ( n =4 or 5). * P <0.05, ** P <0.01, Student’s t -test. ( b ) Flow cytometry in the left panels shows expression of green fluorescent protein (GFP) and Notch2 in cultured podocytes transduced with non-silencing shRNA (control) or three Notch2 shRNAs (N2KD-1, 2, 3). Notch2 expression on the GFP+-transduced cells are indicated as histograms in the lower panels. Percentages of Notch2+ cells in GFP+ cells are also shown (right). ( c ) The podocytes transduced with control shRNA or Notch2 shRNAs were treated with 0.25 μg ml −1 of ADR for 8 h. Percentages of Annexin V+ apoptotic cells in GFP+-transduced cells are indicated as the means±s.e.m. of triplicated cultures. ** P <0.01, Student’s t -test. Full size image Notch2 protects podocytes from apoptosis through Akt pathway To elucidate the mechanisms by which Notch2 protects damaged podocytes from apoptosis, we examined the effect of Notch2 agonistic mAb on anti-apoptotic pathways. Akt pathway is one of the major anti-apoptotic and cell survival pathways that are involved in various organs [23] , [24] , [25] . We found that Notch2 agonistic mAb significantly enhanced ADR-induced activation of Akt, as estimated by phosphorylation at Ser473. Moreover, GSI abrogated the increase of phosphorylation of Akt ( Fig. 5a ). It has been reported that activated Akt promotes cell survival through several pathways, including phosphorylation of pro-apoptotic factors such as Bcl-xL/Bcl-2-associated death (Bad) [23] . Phosphorylated Bad at Ser136 was increased by Notch2 agonistic mAb in parallel with the phosphorylated Akt in podocytes treated with ADR ( Fig. 5b ). Consequently, ADR-induced expression of cleaved caspase-3, one of the final executors of apoptosis, was mostly abolished by Notch2 agonistic mAb ( Fig. 5b ; original results are shown in Supplementary Fig. 4 ). These results suggest that Notch2 protects damaged podocytes from apoptosis possibly through the Akt–Bad pathway. To confirm that Notch2 protects podocytes from apoptosis through the Akt pathway, we next treated ADR-damaged podocytes with triciribine, an inhibitor of Akt phosphorylation, and analysed the effect of triciribine on apoptosis by flow cytometry. The ratio of apoptotic cells in ADR-damaged podocytes increased when triciribine was added ( Fig. 5c ). Futhermore, the protective effect of Notch2 agonistic mAb was abolished by triciribine ( Fig. 5c ), indicating that Notch2 protects podocytes from apoptosis through the Akt pathway. 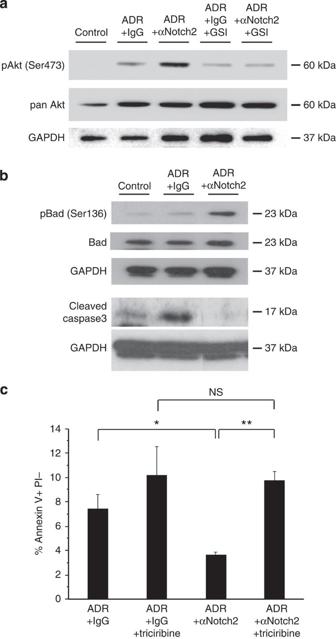Figure 5: Notch2 protects damaged podocytes from apoptosis through Akt pathway. Cultured podocytes were treated with 0.25 μg ml−1ADR and control hamster IgG (IgG) or Notch2 agonistic mAb (αNotch2) in the presence or absence of γ-secretase inhibitor (GSI) for 3 h. The levels of phosphorylated Akt (pAkt) and PAN-Akt (a) and phosphorylated Bad (pBad), Bad and cleaved caspase-3 (b) were assessed by western blotting. (c) The ADR-treated podocytes in the presence of IgG or αNotch2 with/without 20 μM of triciribine were stained with APC-Annexin V/PI at 8 h after the ADR treatment and analysed by flow cytometry. Percentages of Annexin V+ PI− apoptotic cells are indicated as the means±s.e.m. of triplicated cultures. *P<0.05, **P<0.001, Student’st-test. NS, not significant. Figure 5: Notch2 protects damaged podocytes from apoptosis through Akt pathway. Cultured podocytes were treated with 0.25 μg ml −1 ADR and control hamster IgG (IgG) or Notch2 agonistic mAb (αNotch2) in the presence or absence of γ-secretase inhibitor (GSI) for 3 h. The levels of phosphorylated Akt (pAkt) and PAN-Akt ( a ) and phosphorylated Bad (pBad), Bad and cleaved caspase-3 ( b ) were assessed by western blotting. ( c ) The ADR-treated podocytes in the presence of IgG or αNotch2 with/without 20 μM of triciribine were stained with APC-Annexin V/PI at 8 h after the ADR treatment and analysed by flow cytometry. Percentages of Annexin V+ PI− apoptotic cells are indicated as the means±s.e.m. of triplicated cultures. * P <0.05, ** P <0.001, Student’s t -test. NS, not significant. Full size image Notch2 activation correlates with podocyte preservation Lipopolysaccaride (LPS)-induced nephropathy is known as a mouse model of minimal change nephrotic syndrome (MCNS) that does not show podocyte loss [26] . In vitro , treatment of cultured podocytes with LPS increased cleaved Notch2 and activated Akt ( Fig. 6a ), which was partially abrogated by GSI ( Supplementary Fig. 5 ). These results suggest that LPS-induced Akt activation is at least partly mediated by Notch2. In contrast to the ADR-induced nephropathy as an FSGS model, LPS-induced nephropathy was not significantly attenuated by the Notch2 agonistic mAb ( Fig. 6b ). Immunohistological staining showed that almost all podocytes expressed ICN2 at the peak of nephropathy ( Fig. 6c ). These results suggest an association of Notch2 activation with podocyte preservation. 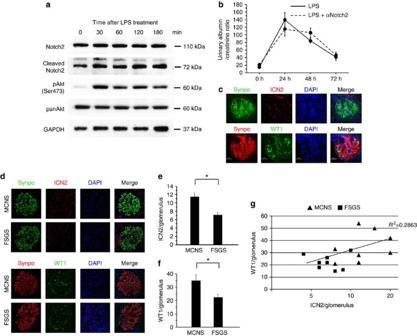Figure 6: Notch2 activation correlates with podocyte preservation in mouse and human glomerular diseases. (a) Time course of Notch2 and Akt activation in LPS-treated podocytes. Cultured podocytes were treated with 50 μg ml−1LPS for the indicated times. (b) Time course assessment of urinary albumin/creatinine ratio in mice injected with LPS. A single dose (200 μg) of LPS with or without Notch2 agonistic mAb (αNotch2) was injected intraperitoneally at 0 h. Urine samples were collected at the indicated hours from at least five mice at each time point. (c) Staining of Synpo, ICN2, WT1 and DAPI in kidney section of mice with LPS nephropathy at 24 h. (d) Staining of Synpo, ICN2, WT1 and DAPI in human kidney biopsy specimens. Kidney samples were pathologically diagnosed. The number of ICN2-positive cells per glomerulus (e) and the number of WT1-positive nucleus per glomerulus (f) are indicated as the means±s.e.m. of eight MCNS and eight FSGS samples. *P<0.05. Student’st-test. (g) Correlation of WT1 and ICN2 was analysed by scatter plot and fitted value (a straight line) is shown. Coefficient of determination is expressed asR2. Figure 6: Notch2 activation correlates with podocyte preservation in mouse and human glomerular diseases. ( a ) Time course of Notch2 and Akt activation in LPS-treated podocytes. Cultured podocytes were treated with 50 μg ml −1 LPS for the indicated times. ( b ) Time course assessment of urinary albumin/creatinine ratio in mice injected with LPS. A single dose (200 μg) of LPS with or without Notch2 agonistic mAb (αNotch2) was injected intraperitoneally at 0 h. Urine samples were collected at the indicated hours from at least five mice at each time point. ( c ) Staining of Synpo, ICN2, WT1 and DAPI in kidney section of mice with LPS nephropathy at 24 h. ( d ) Staining of Synpo, ICN2, WT1 and DAPI in human kidney biopsy specimens. Kidney samples were pathologically diagnosed. The number of ICN2-positive cells per glomerulus ( e ) and the number of WT1-positive nucleus per glomerulus ( f ) are indicated as the means±s.e.m. of eight MCNS and eight FSGS samples. * P <0.05. Student’s t -test. ( g ) Correlation of WT1 and ICN2 was analysed by scatter plot and fitted value (a straight line) is shown. Coefficient of determination is expressed as R 2 . Full size image To investigate whether Notch2 plays a protective role in human glomerular diseases with nephrotic syndrome, we evaluated a correlation between the Notch2 activation and the preservation of podocytes in human specimens of MCNS and FSGS by immunofluorescence study. We performed double staining of WT1, a podocyte nucleus marker, and DAPI to count the number of podocytes accurately. Serial slices of kidney biopsy specimens were used to evaluate a correlation between the expression of cleaved Notch2 (ICN2) and the number of podocytes in each glomerulus. Consistent with a previous report [18] , the expression of ICN2 was decreased in FSGS as compared with that in MCNS ( P =0.0022, Student’s t -test; Fig. 6d,e ). Also, significant loss of podocytes was found in FSGS than in MCNS as previously reported [7] ( P =0.0230, Student’s t -test; Fig. 6d,f ). A positive linear correlation was found between the number of podocytes showing ICN2 and the number of residual podocytes in each glomerulus ( Fig. 6g ). Importantly, glomeruli with MCNS showed more ICN2 and more podocytes (the upper right area in the graph), whereas those with FSGS showed less ICN2 and less podocytes (the lower left area in the graph). Furthermore, less ICN2-positive podocytes tended to be detected in FSGS compared with MCNS even if the number of residual podocytes was equal. Here we demonstrated that Notch2 agonistic mAb ameliorated proteinuria and glomerulosclerosis in a mouse model of nephrosis and FSGS. Our results have revealed that Notch2 pathway plays a critical role in protecting damaged podocytes from apoptosis. Moreover, we have shown a reverse correlation between Notch2 activation and podocyte loss in human glomerular diseases, suggesting a clinical utility of Notch2 agonists to ameliorate nephrosis. The functions of Notch pathway in glomerular diseases remain mostly unclear. So far, two reports evaluated the blockade of Notch pathway using GSI in a rodent model of nephrotic syndrome or genetic engineering in mice [14] , [27] . Interestingly, they demonstrated the opposite results. Niranjan et al . [14] demonstrated that Notch pathway blockade by genetic deletion of Rbpj or by administration of GSI ameliorated the glomerulosclerosis in the mouse model of diabetic nephropathy and the proteinuria in PAN-treated rats. In contrast, Lasagni et al . [27] reported that administration of GSI worsened the proteinuria in ADR nephropathy. The inconsistency of these results might be due to the differences in activated Notch receptor in each disease model. The details about which Notch receptor is activated and which Notch receptor is dominantly involved in each glomerular disease are not completely understood. As we have shown in this study, both Notch1 and Notch2 were activated but their functions were different. They used GSI or genetic deletion of Rbpj in their reports, which interrupts all Notch pathways. It is possible that the consequences might be different when activated Notch pathway was different in each model. Moreover, specific blockade of a particular Notch pathway would lead to different consequences. Our experiments using the agonistic mAb, which specifically interacts with the particular Notch receptor, have revealed that Notch2 pathway is important to recover from damages in podocytes. Hence, Notch2 agonistic mAb can be expected as a new drug for glomerular diseases that specifically works without affecting other Notch pathways. Possible contribution of other cells expressing Notch2 involved in developing kidney diseases such as lymphocytes has not been examined, so further study is needed to address the possibility. The specific role of Notch2 pathway in apoptosis has been demonstrated in some reports, especially in cancer research. Anti-apoptotic function of Notch2 has been reported by Rosati et al . [28] They demonstrated that B-cell chronic lymphoblastic leukaemia showed activation of Notch1 and Notch2, which induced activation of anti-apoptotic molecules such as nuclear factor-κB, cellular inhibitor of apoptosis protein 2 (c-IAP2) and X-linked inhibitor of apoptosis protein (XIAP). They also showed that GSI and Notch2-specific knockdown resulted in apoptosis of B-cell chronic lymphoblastic leukaemia cells. In the present study, we showed possible contribution of the Akt–Bad pathway to the Notch2-mediated protection of podocytes from apoptosis. There are some reports demonstrating the interaction between Notch pathway and Akt pathway [29] , [30] , [31] . Hampel et al . [32] showed the increased phosphorylation of Akt in B cells expressing Notch2 intracellular domain. Our results confirmed the relevance between Notch2 and Akt pathway. We clarified that the podocytes showing Notch2 activation were seen more in MCNS than FSGS by using mouse models and human kidney specimens. Importantly, our data revealed a positive linear correlation between the number of podocytes that activated Notch2 and the number of residual podocytes in a glomerulus in human glomerular diseases. The FSGS glomeruli show less podocytes with activated Notch2 as compared with MCNS. These results suggest that the less activation of Notch2 in podocytes might result in the podocyte loss in FSGS. Although Notch2 agoinistic mAb dramatically reduced proteinuria in ADR nephropathy, it did not affect proteinuria in LPS nephropathy. We assume that Notch2 mAb did not induce further activation of Notch2 because sufficient activation of Notch2 was achieved endogeneously in LPS nephropathy. We showed that Notch2–Akt pathway is induced by LPS as well as by ADR in vitro . However, it is known that Toll-like receptor 4 is activated by LPS, leading to the activation of Akt. Thus, Toll-like receptor 4-mediated Akt activation might also contribute to the protection of podocytes in this LPS-induced model. Notch pathway has a potential to have interactions with other specific molecules and pathways involved in MCNS and FSGS. Soluble urokinase receptor (suPAR), reported as a cause of FSGS [33] , is one of those. There is a report demonstrating that downregulation of uPAR inhibits the cleavage of Notch1 receptor and the gene expression of Notch1 mRNA [34] . Wei et al . [33] have shown that suPAR causes proteinuria and FSGS-like glomerulopathy. Therefore, it is possible that suPAR and Notch1 have an interaction leading to podocyte injury. This possibility would be one of the future subjects to explore. Another candidate molecule that might have interactions with Notch pathway and be involved in podocyte injury is dendrin. Previous studies from our lab demonstrated the relocation of dendrin from the slit diaphragm to the podocyte nucleus, leading to apoptosis of podocytes [22] . Notch2 has a role to prevent apoptosis of podocytes. Thus, there is a possibility that Notch2 pathway may prevent relocation of dendrin into nucleus in podocytes. In addition, it is notable that MCNS shows more activated Notch2 in podoccytes in vivo . Recently, Clement et al . [35] showed that angiopoietin-like 4 had a key role to cause MCNS. It is possible that Notch2 may have a function to suppress the angiopoietin-like 4 expression. Further studies are needed to clarify the interaction of Notch2 pathway with these known pathways for MCNS and FSGS. Taken together, acceleration of Notch2 activation by using agonistic mAb has a potential to rescue damaged podocytes and prevent the progression of glomerulosclerosis in human glomerular diseases. Mouse models This study was conducted according to the Declaration of Helsinki and was approved by Institutional Review Board of Juntendo University. Female BALB/c mice were purchased from Oriental Yeast Co., Ltd. (Tokyo, Japan). ADR-induced nephropathy was conducted [22] . In brief, ADR (doxorubicin hydrochloride; Wako, Osaka, Japan) diluted with 0.9% saline at a dose of 10 mg kg −1 body weight was injected once to BALB/c mice at 6 weeks of age via the tail vein. Age-matched control mice were injected with an equal volume of PBS. The Jagged1 antagonistic mAb (HMJ1-29), Notch1 agonistic mAb (HMN1-12) and Notch2 agonistic mAb (HMN2-29) were generated and characterized. To generate Jagged1 antagonistic mAb, Chinese hamster ovary (CHO) cells expressing murine Jagged1 were prepared. Armenian female hamsters at 6 weeks of age (Oriental Yeast) were immunized by intraperitoneal injection of Jagged1-expressing CHO cells three times at 7-day intervals. Three days after the final immunization, the splenocytes were fused with P3U1 myeloma cells. After HAT selection, antibodies that reacted Jagged1-transfected CHO cells, but not with untransfected CHO cells, were screened by flow cytometry. Each mAb was cloned by limiting dilution. To generate the mAbs that react with mouse Notch1 or Notch2, Armenian hamsters were immunized by intraperitoneal injection of mouse Notch1- or Notch2-Fc fusion proteins three times at 7-day intervals. The hybridoma cells were prepared as described above, and antibodies that reacted with mouse Notch2-transfected CHO cells, but not with untransfected CHO cells, were screened and cloned. All these mAbs were purified from ascites produced in pristan-primed ICR nude mice by the caprylic acid and ammonium sulphate precipitation method [36] , [37] , [38] , [39] . Two hundred and fifty micrograms of HMJ1-29 or control hamster IgG (UC8-1B9) and 100 μg of HMN1-12 or HMN2-29 were injected intraperitoneally on the indicated days. A single dose (200 μg) of LPS purchased from Sigma-Aldrich (MI, USA) was intraperitoneally injected to BALB/c mice to generate LPS-induced nephropathy. Control IgG or HMN2-29 (100 μg) were intraperitoneally injected just before LPS. Renal histology and immunohistochemistry The kidneys of female mice at 6–10 weeks of age were fixed by perfusion of 4% paraformaldehyde and 20% sucrose in PBS, and embedded in paraffin for light microscopic study. For the histological study, 3-μm sections were stained by the periodic acid–Schiff method. The sections were observed under light microscopy (Olympus BX41; Olympus, Tokyo, Japan). For immunofluorescence study, the fixed kidneys were frozen in optimal cutting temperature compound. Frozen sections (4–5 μm) were incubated with primary antibodies specific for cleaved Notch1 (Val1744; #2421; Cell Signaling, MA, USA), cleaved Notch 2 (anti-Notch2 antibody, amino terminus, 07-1234; Millipore, MA, USA), synaptopodin (65194; Progen, Heidelberg, Germany) or WT1 (SC-192; Santa Cruz, CA, USA), and developed with secondary antibodies. The human kidney specimens were fixed with 4% paraformaldehyde and 2% sucrose in PBS and frozen sections were immunostained in the same way. Biochemical analyses of urine samples Urinary albumin to creatinine ratio was measured using an immunoassay (DCA 2000 Systems; SIEMENS, Munich, Germany) with a Bayer DCA 2000+ chemical analyser (Bayer, Leverkusen, Germany). Cell culture and transfection of podocytes Conditionally immortalized mouse podocytes were cultured in RPMI-1640 cell medium (Sigma or Wako) containing 10% FBS, penicillin/streptomycin (Life Technologies, CA, USA) and interferon-γ (10 U ml −1 ) at 33 °C. Podocytes were incubated at 37 °C for 10–14 days to differentiate [40] . To inhibit Notch pathway, 10 μM of GSI (Calbiochem, Darmstadt, Germany) was added to [41] cultured podocytes. To generate N2KD podocytes, we used GIPZ lentiviral shRNA system (Thermo Scientific, MA, USA) following the manufacturer’s instructions. In brief, HEK293T cells were transfected with shRNA plasmid DNA (GIPZ non-silencing lentiviral shRNA control as a control, V2LMM_226932 as N2KD-1, V3LMM_483503 as N2KD-2 or V3LMM_483503 as N2KD-3) to produce lentiviral particles. Differentiated cultured podocytes were transduced with the lentiviral particles and the transduction was confirmed by flow cytometry detecting GFP (green fluorescent protein). Podocytes were treated with 0.25 μg ml −1 of ADR to induce cell damage, with/without 50 μg ml −1 of HMN2-29 or UC8-1B9. To inhibit Akt pathway, 20 μM of triciribine (Merck KGaA, Darmstadt, Germany) was added. To investigate the effect of LPS, podocytes were treated with 50 μg ml −1 of LPS. Western blotting In brief, cells were lysed in 1% Triton buffer. Samples were resolved on SDS–polyacrylamide gels. The gels were transferred to membrane and blocked with 5% non-fat milk. The membranes were incubated with the appropriate primary antibodies. Primary antibodies were detected by binding horseradish peroxidase-conjugated secondary antibody with detection reagents. Primary antibodies: Notch2 (D76A6) (#5732), Jagged1 (28H8) (#2620), phospho-Akt (Ser473) (D9E) (#4060), Akt (PAN) (C67E7) (#4691), phospho-Bad (Ser136) (D25H8) (#4366), Bad (D24A9) (#9239) and cleaved caspase-3 (Asp175) (#9661) were purchased from Cell Signaling, and anti-Notch2 antibody, N terminus (07-1234) were purchased from Millipore. These primary antibodies were used at 1:1,000 dilution for western blotting. Primary antibody for GAPDH (G8795) was purchased from Sigma-Aldrich and used at 1:10,000 dilution. Cytotoxicity assay Cytotoxicity at 48 h in podocytes was measured by the LDH release assay. LDH activity in cultured supernatants was assessed with Cytotoxicity Detection Kit PLUS (Roche, Basel, Switzerland) following the manufacturer’s instructions. One percent Triton was used to lyse all cells. Apoptosis assay Apoptotic cells were identified by staining with allophycocyanin (APC)-labelled annexin V and propidium iodide [42] by using Annexin V Apoptosis Detection Kit APC (eBioscience, CA, USA). The cells were collected at 8 h after ADR treatment, washed and suspended in the binding solution. APC-annexin V was added at dilutions recommended by the manufacturer. After 10 min, the cells were washed and suspended in the binding solution, and then PI was added. At least 10,000 cells per sample were analysed on FACS Calibur (BD) and data were analysed using CellQuest Pro software (BD). Apoptotic cells were identified as the annexin V+ PI− cells. Real-time PCR Total RNAs from cultured podocytes was extracted using the RNeasy Mini Kit (Qiagen, Hieden, Germany). The amount of RNA was determined and total RNA was reverse transcribed using either M-MuLVRT (Promega, WI, USA) or SuperscriptIII (Life Technologies) for first-strand complementary DNA. Real-time PCR assays were performed using TaqMan Real-Time PCR Assays (TaqMan Fast Advanced Master Mix 4444557, jagged 1 Mm00496902_m1, notch 2 Mm00803077_m1, hairy and enhancer of split 1 (Drosophila) Mm01342805_m1, hairy and enhancer of split 5 (Drosophila) Mm00439311_g1, hairy/enhancer-of-split related with YRPW motif 1 Mm00468865_m1, hairy/enhancer-of-split related with YRPW motif-like Mm00516555_m1 and glyceraldehyde-3-phosphate dehydrogenase Mm99999915_g1; Life Technologies) and 7,500 real-time PCR system (Life Technologies), following the manufacturer’s instructions. All measured values were normalized with glyceraldehyde-3-phosphate dehydrogenase and calculated using the ΔΔCT method. Statistical analysis Quantification of western blotting was performed with image processing software (imageJ). Data are represented as the mean±s.e.m. Student’s t -test was used to analyse the difference between two groups. Values were regarded significant at P <0.05. Human kidney specimens Human kidney specimens were collected from kidney biopsies that were performed at the Juntendo University Hospital, Tokyo, Japan. This study was conducted according to the Declaration of Helsinki and was approved by Institutional Review Board of Juntendo University Hospital. Informed consent was obtained from all patients. We selected the cases that developed nephrotic syndrome and that were proven to be MCNS and FSGS. Three patients in each group were examined. How to cite this article: Tanaka, E. et al . Notch2 activation ameliorates nephrosis. Nat. Commun. 5:3296 doi: 10.1038/ncomms4296 (2014).